Septins promote dendrite and axon development by negatively regulating microtubule stability via HDAC6-mediated deacetylation Neurite growth requires two guanine nucleotide-binding protein polymers of tubulins and septins. However, whether and how those cytoskeletal systems are coordinated was unknown. Here we show that the acute knockdown or knockout of the pivotal septin subunit SEPT7 from cerebrocortical neurons impairs their interhemispheric and cerebrospinal axon projections and dendritogenesis in perinatal mice, when the microtubules are severely hyperacetylated. The resulting hyperstabilization and growth retardation of microtubules are demonstrated in vitro . The phenotypic similarity between SEPT7 depletion and the pharmacological inhibition of α-tubulin deacetylase HDAC6 reveals that HDAC6 requires SEPT7 not for its enzymatic activity, but to associate with acetylated α-tubulin. These and other findings indicate that septins provide a physical scaffold for HDAC6 to achieve efficient microtubule deacetylation, thereby negatively regulating microtubule stability to an optimal level for neuritogenesis. Our findings shed light on the mechanisms underlying the HDAC6-mediated coupling of the two ubiquitous cytoskeletal systems during neural development. The organization of the neural network depends on two distinct types of subcellular protrusions, dendrites and axons. Despite the diversity in morphology, composition and function, all neurites share a common structural backbone, the microtubule. The assembly and the balance between the dynamic instability and stability of microtubules are under multiplex control [1] . However, among the plethora of proteins that associate with microtubules, only a fraction of them has been assigned to physiological molecular pathways that control microtubules during neuritogenesis [2] . Genetic studies have indicated that neuritogenesis in nematodes requires septins [3] , [4] , a family of heteropolymerizing guanosine tri-/di-phosphate-binding proteins whose mammalian homologues associate with microtubules in the brain [5] . Although septin-null nematodes exhibit complex phenotypes, including neurite anomalies and uncoordinated locomotor defects [6] , a fundamental question remains as to whether the neurological defects are direct, or even cell autonomous, consequences due to the loss of septins. Attempts with mouse reverse genetics so far have failed to provide informative findings as to whether and how mammalian septins (SEPT1–14) are required for neuritogenesis in vivo . The genetic disruption of one or two functionally redundant subunits within the septin family (that is, SEPT3, SEPT4, SEPT5, SEPT6, SEPT3 and SEPT5, or SEPT4 and SEPT6) gives no recognizable morphological anomaly in the nervous system, partly due to the adaptive upregulation of functionally similar subunits and/or other modes of compensation [7] , [8] , [9] , [10] , [11] . In contrast, embryos that lack the uniquely nonredundant subunit SEPT7 collapse by midgestation [12] . Mosaic analysis might offer a means to overcome the limitations of genetic approaches to characterize the redundant and multifunctional system of septins. We hypothesized that either local gene disruption or local acute depletion of a pivotal septin subunit from postmitotic, sprouting neurons might reveal a phenotype that is otherwise masked. A reasonable strategy would be to probe neuritogenesis in the developing brain via the local depletion of SEPT7 on the basis of the following evidence obtained in vitro : First, acute depletion of SEPT7 via RNA interference (RNAi) causes collateral destabilization and reduction of other subunits that constitute hetero-oligomers, which abolishes the entire septin system in mouse T lymphocytes [13] . Second, RNAi-mediated depletion of SEPT7 from rat hippocampal neurons in dissociation culture perturbs dendrite development, although the molecular mechanism and in vivo relevance of that phenomenon are unknown [14] , [15] . The present study is designed for the parallel examination of in vivo and in vitro phenotypes of postmitotic cerebrocortical neurons after local and acute depletion of SEPT7 via RNAi or conditional gene disruption via the Cre-loxP recombination system. This approach reveals obvious neuritogenesis defects in vivo for the first time in vertebrates, and enables us to further investigate this mechanism in neurons dissociated in vitro , an experimental system which is more amenable to rigorous morphometry, molecular pharmacology, in situ antibody crosslinking assays and live imaging. Our combined approach allows us to uncover a novel septin-null phenotype in developing mouse brain, an unexpected mode of interaction between the microtubule and septin cytoskeletal systems, and a novel septin scaffold-based regulatory mechanism of HDAC6 as a deacetylase/adapter of α/β-tubulins. We conclude that neuronal septins provide a scaffold for the efficient microtubule deacetylation by HDAC6, which optimizes the growth and stability of microtubule for neuritogenesis during pre- and postnatal development of mammalian brain. SEPT7 is required for neuritogenesis in the mouse brain Previous in vitro studies have shown that primary neurons cultured from rat hippocampus and from the chick dorsal root ganglion require septins for dendrite development [14] , [15] and axon branching [16] , respectively. To test the relationship and in vivo relevance of those findings and to explore the molecular mechanism(s) involved, we employed mouse cerebrocortical neurons, which enable both physiological analyses in vivo and rigorous morphometry and live imaging in vitro [17] , [18] , [19] . By immunoprecipitation and immunoblot analyses, we found that perinatal mouse cerebrocortical neurons express most of the septin subunits in vivo and in vitro as do rat hippocampal neurons [15] , and that SEPT5, SEPT6, SEPT7 and SEPT11 constitute the major septin species that form hetero-oligomers ( Supplementary Fig. S1 ). To perturb the septin system, the pivotal subunit SEPT7 was depleted by expressing two distinct shRNAs against Sept7 , when GFP was co-expressed as a marker of transfection and cell volume for morphometry [20] . The efficiency of SEPT7 depletion was ~80% determined by immunofluorescence of GFP-positive cerebrocortical neurons electroporated and cultured in vitro ( Fig. 1a ) and by immunoblot of FACS-fractionated GFP-positive cerebrocortical neurons that had been electroporated in utero ( Fig. 1b and Supplementary Fig. S2 ). 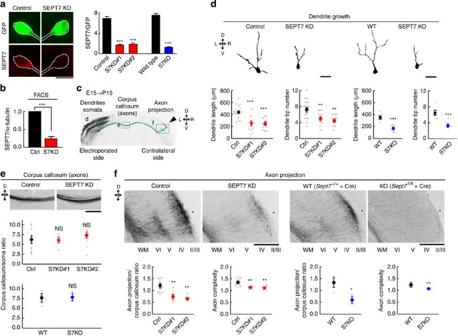Figure 1: The core septin subunit SEPT7 is required for the growth of dendrites and axons of cerebrocortical neuronsin vivo. (a) Representative immunofluorescence images of primary cerebrocortical neurons at div2 co-expressing GFP with control (left) or shRNA#1 against SEPT7 (right). Endogenous SEPT7 (red) is depleted in GFP-positive transfectants (green). Scale bar, 10 μm. Graph: SEPT7 depletion efficiency (SEPT7/GFP immunofluorescence ratio) via RNAi (S7KD#1, #2) or acute gene disruption (S7KO). (n=12. ***P<0.001 by one-way ANOVA withpost hocTukey for KD,t-test for KO). Error bars denote s.e.m. (b) SEPT7 depletion efficiency (SEPT7/α-tubulin immunofluorescence ratio)in vivovia RNAi (S7KD#1). FACS-sorted GFP-positive neurons from P2 cerebral cortices were immunoblotted. Triplicated experiments. (***P<0.001 byt-test. SeeSupplementary Fig. S2). Error bars denote s.e.m. (c) P15 mouse coronal section with a layer II/III pyramidal neuron in the somatosensory cortex (S1/S2). Prospective layer II/III pyramidal neurons were subjected to KD/KO at E15 and analysed at P15 for the dendrites (d), callosal axon bundles (e) and axon terminals in the contralateral S1/S2 (f). (d) Representative projected images of GFP-positive layer II/III pyramidal neurons. Scale bars, 50 μm. Graph: SEPT7 depletion via KD/KO consistently reduced the total length and tip number of dendrites. (KD;n=18, 12, 12. ***P<0.001 by one-way ANOVA withpost hocTukey. KO;n=7, ***P<0.001,t-test). Error bars denote s.e.m. (e) Representative images of GFP-positive axon bundles at the corpus callosum. Scale bar, 250 μm. Graph: SEPT7 depletion did not affect the axon projection up to the midline. (KD;n=12, 6, 6. NS,P>0.05 by one-way ANOVA withpost hocTukey. KO;n=3. NS,P>0.05 byt-test). Error bars denote s.e.m. (f) Representative images of GFP-positive axon terminals projecting toward the contralateral S1/S2 (asterisk). The axon terminals branch and terminate at layers V and II/III. Layers (II/III to VI) and white matter (WM) are labelled at the bottom. Scale bars, 500 μm. Graph: GFP-fluorescence intensity in layers II/III normalized to the corpus callosum and the axon complexity at a distal segment (the ratio of the number of branches that entered layer IV over that at layer V) were significantly diminished in SEPT7-depleted neurons. Thus, the terminal extension and branching of axons were consistently impaired via RNAi and gene disruption. (KD;n=12, 6, 6. **P<0.01 by one-way ANOVA withpost hocTukey. KO;n=3. **P<0.01, *P<0.05 byt-test). Error bars denote s.e.m. Figure 1: The core septin subunit SEPT7 is required for the growth of dendrites and axons of cerebrocortical neurons in vivo . ( a ) Representative immunofluorescence images of primary cerebrocortical neurons at div2 co-expressing GFP with control (left) or shRNA#1 against SEPT7 (right). Endogenous SEPT7 (red) is depleted in GFP-positive transfectants (green). Scale bar, 10 μm. Graph: SEPT7 depletion efficiency (SEPT7/GFP immunofluorescence ratio) via RNAi (S7KD#1, #2) or acute gene disruption (S7KO). ( n =12. *** P <0.001 by one-way ANOVA with post hoc Tukey for KD, t -test for KO). Error bars denote s.e.m. ( b ) SEPT7 depletion efficiency (SEPT7/α-tubulin immunofluorescence ratio) in vivo via RNAi (S7KD#1). FACS-sorted GFP-positive neurons from P2 cerebral cortices were immunoblotted. Triplicated experiments. (*** P <0.001 by t -test. See Supplementary Fig. S2 ). Error bars denote s.e.m. ( c ) P15 mouse coronal section with a layer II/III pyramidal neuron in the somatosensory cortex (S1/S2). Prospective layer II/III pyramidal neurons were subjected to KD/KO at E15 and analysed at P15 for the dendrites ( d ), callosal axon bundles ( e ) and axon terminals in the contralateral S1/S2 ( f ). ( d ) Representative projected images of GFP-positive layer II/III pyramidal neurons. Scale bars, 50 μm. Graph: SEPT7 depletion via KD/KO consistently reduced the total length and tip number of dendrites. (KD; n =18, 12, 12. *** P <0.001 by one-way ANOVA with post hoc Tukey. KO; n =7, *** P <0.001, t -test). Error bars denote s.e.m. ( e ) Representative images of GFP-positive axon bundles at the corpus callosum. Scale bar, 250 μm. Graph: SEPT7 depletion did not affect the axon projection up to the midline. (KD; n =12, 6, 6. NS, P >0.05 by one-way ANOVA with post hoc Tukey. KO; n =3. NS, P >0.05 by t -test). Error bars denote s.e.m. ( f ) Representative images of GFP-positive axon terminals projecting toward the contralateral S1/S2 (asterisk). The axon terminals branch and terminate at layers V and II/III. Layers (II/III to VI) and white matter (WM) are labelled at the bottom. Scale bars, 500 μm. Graph: GFP-fluorescence intensity in layers II/III normalized to the corpus callosum and the axon complexity at a distal segment (the ratio of the number of branches that entered layer IV over that at layer V) were significantly diminished in SEPT7-depleted neurons. Thus, the terminal extension and branching of axons were consistently impaired via RNAi and gene disruption. (KD; n =12, 6, 6. ** P <0.01 by one-way ANOVA with post hoc Tukey. KO; n =3. ** P <0.01, * P <0.05 by t -test). Error bars denote s.e.m. Full size image To test whether SEPT7 is required for neuritogenesis in a physiological context, we first focused on the perinatal development of pyramidal neurons in layer II/III of the primary and secondary somatosensory cortex (S1/S2). Each neuron emanates several dendrites apically and an axon basally to deeper layers, and the axon traverses the corpus callosum and projects towards layers II/III/V of the contralateral S1/S2. We injected two different sh Sept7 /GFP plasmids with distinct target sequences (#1 and #2) into the left lateral ventricle beneath the left S1/S2 of E15 embryos in utero , and conducted electroporation targeting pyramidal neuron precursors destined to undergo radial migration to layer II/III. The migration, dendrite growth and interhemispheric axon projection of pyramidal neurons are known to complete by P15, when we conducted morphological analyses with coronal brain sections ( Fig. 1c ). We confirmed that local depletion of SEPT7 by either of those short hairpin RNAs (shRNAs) did not affect either the survival of neurons or their radial migration toward layer II/III ( Supplementary Fig. S3 ). However, morphometry of GFP-positive pyramidal neurons in layer II/III of ipsilateral S1/S2 demonstrated statistically significant reductions in the total length and complexity (that is, branch tip number) of dendrites projecting locally from SEPT7-depleted neurons as compared with the control ( Fig. 1d , left). As morphometry was not applicable for individual axons in bundles, we measured the fluorescence intensity of the three neuronal segments; dendrites/somata at the ipsilateral S1/S2 layer II/III, the axon bundle at the corpus callosum and axon terminals at the contralateral S1/S2 layer II/III/V ( Fig. 1c ). The ratio of fluorescence intensity at the corpus callosum over that at dendrites/somata was comparable with or without SEPT7 depletion ( Fig. 1e , top), indicating that depletion of SEPT7 does not significantly affect the axon projection up to the corpus callosum. In contrast, the ratio of fluorescence intensities and the branch numbers at the axon terminals over the fluorescence intensity at the corpus callosum was significantly reduced by depletion of SEPT7 ( Fig. 1f , left), indicating defective extension and branching at the distal parts of axons. A follow-up observation at P30 corroborated that none of the morphological abnormality was corrected by weaning ( Supplementary Fig. S4 ), indicating that perinatal depletion of SEPT7 causes irreversible defects in dendritogenesis and axonogenesis. Further, electroporation at an earlier stage (E12) into another subset of neurons to form the primary motor cortex (M1) impaired the corticospinal tract development by affecting the axon projection from the layer V primary motor neurons ( Supplementary Fig. S5 ). To corroborate the findings obtained from the RNAi experiments, we disrupted the Sept7 gene by creating mice harbouring a Cre-loxP-based conditional knockout (floxed) allele, Sept7 fl . Two days after the co-transfection of expression plasmids for Myc-Cre and GFP (as a morphological tracer) into Sept7 fl/fl cerebrocortical neurons, the efficiency of SEPT7 depletion was ~80% determined by the immunofluorescence of cerebrocortical neurons electroporated in vitro ( Fig. 1a , right). We confirmed the comparable effects of SEPT7 depletion on dendrite growth, interhemispheric axon projection and terminal branching of layer II/III pyramidal neurons in S1/S2 ( Fig. 1d , right; 1e, bottom; 1f, right). Together, these data consistently indicate that SEPT7 is commonly required for the elongation and branching of both dendrites and axons in the developing mouse brain. This is the first evidence for the cell autonomous requirement of septins in neuritogenesis in vivo . SEPT7 is required for dendrito- and axonogenesis in vitro To rigorously assess the short dendrite/axon phenotype, we quantified the effects of SEPT7 depletion from cerebrocortical neurons via RNAi or gene disruption in vitro . Two days after transfection of the sh Sept7 /GFP plasmid, the gross knockdown efficiency estimated by immunoblot for SEPT7 (including the GFP-negative population of 30–40%) was ~30–40% ( Fig. 2a and Supplementary Fig. S10 ), whereas the knockdown efficiency per individual GFP-positive cell estimated by immunofluorescence for SEPT7 was ~80% ( Fig. 1a ). Each of the SEPT7-depleted pyramidal-like neurons typically bore several dendrites and an axon as did the control neurons ( Fig. 2b ). Morphometry that separately quantified the total lengths of dendrites and the axon of each neuron revealed that SEPT7-depleted pyramidal-like neurons bore significantly shorter dendrites (60 versus 105 μm at the 50th percentile) and axons (210 versus 350 μm at the 50th percentile) with less complexity (branch tip number) than the control. Scattergram analysis indicates that depletion of SEPT7 caused proportional defects in dendrites and axons in individual neurons. The morphological phenotype was almost completely rescued by co-expressing an RNAi-resistant Sept7 mRNA with a red fluorescent protein, mCherry ( Fig. 2c,d ). 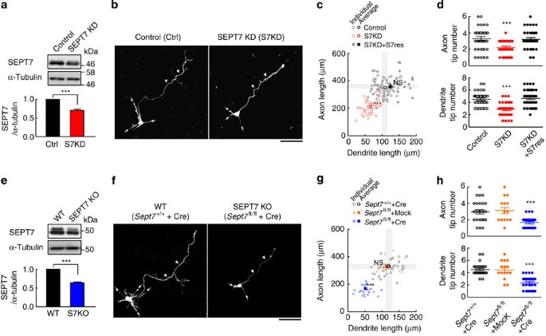Figure 2:In vitrorescue and morphometry of the SEPT7-depletion phenotype on dendrite/axon growth. (a) Immunoblot estimation of the gross efficiency (including GFP-negative untransfected population) of SEPT7 depletion from wild-type E17 embryo-derived neurons via S7KD#1 RNAi (div2). Each lane contained 10 μg protein. (Triplicated experiments. ***P<0.001 byt-test). Error bars denote s.e.m. (b) Representative images for the morphometry of GFP-positive pyramidal-like neurons with dendrites (arrows) and axons (arrowheads). Scale bar, 50 μm. (c) Scattergram of the total lengths of the axon and dendrites from each neuron expressing the designated plasmid(s). Dendrites and axons of SEPT7-depleted neurons (S7KD, red) were significantly and proportionally shorter than control neurons (black) whose average±2 s.e.m. is indicated as grey zones. The SEPT7-depletion phenotype was rescued by the co-expression of an RNAi-resistant mRNA encoding mCherry-SEPT7 (S7KD+S7res, closed circles). (n=45 × 3. ***P<0.001; NS,P>0.05 by one-way ANOVA withpost hocTukey). Error bars denote s.e.m. (d) Significant differences in the tip numbers of axons and dendrites between the experimental groups (n=45 × 3. ***P<0.001 by one-way ANOVA withpost hocTukey), which were rescued as noted above. Error bars denote s.e.m. (e) Experiment comparable with (a), but usingSept7fl/flembryo and Myc-Cre plasmid. Immunoblot estimation of the gross efficiency (including the untransfected population) of SEPT7 depletion after gene disruption (div2). See legend in (a). Error bars denote s.e.m. (f) Representative images for the morphometry of GFP/Cre-positive,Sept7+/+/wild type (WT) andSept7fl/fl(SEPT7KO) pyramidal-like neurons. See legend in (b). (g) Scattergram of the total lengths of the axon and dendrites from each neuron with designated genotype ±Cre expression. Dendrites and axons ofSept7fl/fl+Cre (SEPT7KO, blue circles) neurons were significantly and proportionally shorter than those of controlSept7fl/fl−Cre (orange circles) neurons andSept7+/++Cre (open circles) neurons whose average±2s.e.m. is indicated as grey zones. Statistical analysis showed that acuteSept7disruption significantly and proportionally shortened their dendrites and axons. (n=30, 15, 30. ***P<0.001 by one-way ANOVA withpost hocTukey). Note that the short dendrite/axon phenotype elicited by gene disruption was more severe than elicited by RNAi in (c). Error bars denote s.e.m. (h) The tip numbers of axons and dendrites were significantly reduced afterSept7disruption. (n=30, 15, 30. ***P<0.001 by one-way ANOVA withpost hocTukey). Error bars denote s.e.m. Figure 2: In vitro rescue and morphometry of the SEPT7-depletion phenotype on dendrite/axon growth. ( a ) Immunoblot estimation of the gross efficiency (including GFP-negative untransfected population) of SEPT7 depletion from wild-type E17 embryo-derived neurons via S7KD#1 RNAi (div2). Each lane contained 10 μg protein. (Triplicated experiments. *** P <0.001 by t -test). Error bars denote s.e.m. ( b ) Representative images for the morphometry of GFP-positive pyramidal-like neurons with dendrites (arrows) and axons (arrowheads). Scale bar, 50 μm. ( c ) Scattergram of the total lengths of the axon and dendrites from each neuron expressing the designated plasmid(s). Dendrites and axons of SEPT7-depleted neurons (S7KD, red) were significantly and proportionally shorter than control neurons (black) whose average±2 s.e.m. is indicated as grey zones. The SEPT7-depletion phenotype was rescued by the co-expression of an RNAi-resistant mRNA encoding mCherry-SEPT7 (S7KD+S7res, closed circles). ( n =45 × 3. *** P <0.001; NS, P >0.05 by one-way ANOVA with post hoc Tukey). Error bars denote s.e.m. ( d ) Significant differences in the tip numbers of axons and dendrites between the experimental groups ( n =45 × 3. *** P <0.001 by one-way ANOVA with post hoc Tukey), which were rescued as noted above. Error bars denote s.e.m. ( e ) Experiment comparable with ( a ), but using Sept7 fl/fl embryo and Myc-Cre plasmid. Immunoblot estimation of the gross efficiency (including the untransfected population) of SEPT7 depletion after gene disruption (div2). See legend in ( a ). Error bars denote s.e.m. ( f ) Representative images for the morphometry of GFP/Cre-positive, Sept7 +/+ /wild type (WT) and Sept7 fl/fl (SEPT7KO) pyramidal-like neurons. See legend in ( b ). ( g ) Scattergram of the total lengths of the axon and dendrites from each neuron with designated genotype ±Cre expression. Dendrites and axons of Sept7 fl/fl +Cre (SEPT7KO, blue circles) neurons were significantly and proportionally shorter than those of control Sept7 fl/fl −Cre (orange circles) neurons and Sept7 +/+ +Cre (open circles) neurons whose average±2s.e.m. is indicated as grey zones. Statistical analysis showed that acute Sept7 disruption significantly and proportionally shortened their dendrites and axons. ( n =30, 15, 30. *** P <0.001 by one-way ANOVA with post hoc Tukey). Note that the short dendrite/axon phenotype elicited by gene disruption was more severe than elicited by RNAi in ( c ). Error bars denote s.e.m. ( h ) The tip numbers of axons and dendrites were significantly reduced after Sept7 disruption. ( n =30, 15, 30. *** P <0.001 by one-way ANOVA with post hoc Tukey). Error bars denote s.e.m. Full size image The findings obtained from the RNAi experiments were corroborated by Sept7 gene disruption. Two days after the co-expression of Myc-Cre and GFP into Sept7 fl/fl cerebrocortical neurons, SEPT7 depletion estimated by immunoblot analysis was ~50% (including a GFP-negative population of 30–40%) ( Fig. 2e and Supplementary Fig. S10 ), when Sept7 -null pyramidal-like neurons bore significantly shorter dendrites (53 versus 120 μm at the 50th percentile) and axons (168 versus 328 μm at the 50th percentile) with less complexity than the control ( Fig. 2f–h ). The possibility of Cre-mediated toxicity on neuritogenesis was excluded by control wild-type neurons expressing Cre. Taken together, the consistent growth impairment of dendrites and axons after the acute partial depletion of SEPT7, either in vivo or in vitro , either via RNAi or gene disruption, indicates the physiological requirement of SEPT7 in a common cell autonomous mechanism that drives neurite extension. SEPT7 limits acetylation and stabilization of microtubules One of the common and major structural determinants of dendritogenesis and axonogenesis is the dynamic assembly of microtubules, which is regulated by a number of mechanisms including tubulin modifications [21] . On the basis of previous studies on aberrant microtubule modifications in septin-depleted non-neural cells (see Discussion), we examined the status of the two major microtubule modifications, acetylation and polyglutamylation, in cerebrocortical neurons in vivo and in vitro . Acetylated α-tubulin significantly accumulated in GFP-positive/SEPT7-depleted layer II/III cerebrocortical neurons, determined by immunoblot of FACS-collected neurons from E17 embryos ( × 5, Fig. 3a and Supplementary Fig. S10 ), and by immunofluorescence of the somata and dendrites ( × 9, Fig. 3b ) and of axons to a lesser extent ( × 3, Fig. 3c ). The differential acetylation levels of dendrites and axons might be correlated with the differential effects of SEPT7 depletion observed in vivo ( Fig. 1d,f ). 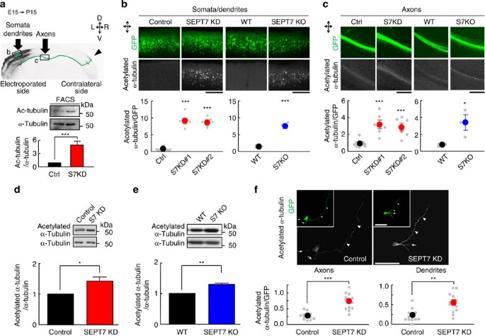Figure 3: Depletion of SEPT7 causes significant accumulation of acetylated α-tubulinin vivoandin vitro. (a) (top) Coronal section of P15 brain depicting two subcellular segments of layer II/III pyramidal neurons in S1/S2 (modified fromFig. 1c). (bottom) FACS-sorted GFP-positive cerebrocortical neurons electroporatedin uteroat E15 and collected at P2 (Supplementary Fig. S2) were immunoblotted for total and acetylated α-tubulin. Depletion of SEPT7 by RNAi caused significant acetylation of α-tubulin. (Triplicated experiments. ***P<0.001 byt-test). Error bars denote s.e.m. (b,c) Image-based quantification of acetylated α-tubulin in the somata and dendrites and the axon bundle proximal to the corpus callosum. (top) Representative immunofluorescence images of acetylated α-tubulin in the somata/dendrites (b) and in the axon bundle (c) of GFP-positive S1/S2 pyramidal neurons with or without SEPT7 depletion via RNAi (#1) or gene disruption. In SEPT7-depleted neurons, microtubules were significantly acetylated in the somata/dendrites and in the axons to a lesser extent. Scale bars, 500 μm (b), 200 μm (c). Graphs: Acetylated α-tubulin/GFP immunofluorescence ratioin vivovia RNAi (S7KD#1 and #2) or gene disruption (S7KO). All three modes of SEPT7 depletion consistently caused significant acetylation of α-tubulin in the somata/dendrites and in the axons to a lesser extent. (KD;n=12, 6, 6. ***P<0.001 by one-way ANOVA withpost hocTukey. KO;n=3, ***P<0.001, *P<0.05 byt-test). Error bars denote s.e.m. (d,e) Immunoblot estimation of the gross acetylated/total α-tubulin ratio (including GFP-negative untransfected population) in SEPT7-depleted cerebrocortical neurons via RNAi (#1, KD) or gene disruption (KO) at div2. Note that α-tubulin was hyperacetylated in SEPT7-depleted neurons. (Triplicated experiments. *P<0.05, **P<0.001 byt-test). Error bars denote s.e.m. (f) (top) Representative immunofluorescence images of acetylated α-tubulin in pyramidal-like cerebrocortical neurons in culture (div2). The insets show GFP co-expressed with shSept7(#1) or the empty vector. The signals for acetylated α-tubulin were elevated in the soma, dendrites and axons of SEPT7-depleted neurons (SEPT7 KD). Scale bars, 50 μm. (bottom) Quantification of acetylated α-tubulin immunofluorescence measured separately in dendrites and axons, showing that SEPT7 depletion caused hyperacetylation of microtubules in axons and dendrites to a comparable degree. (n=12, ***P<0.001, **P<0.01 byt-test). Error bars denote s.e.m. Figure 3: Depletion of SEPT7 causes significant accumulation of acetylated α-tubulin in vivo and in vitro. ( a ) (top) Coronal section of P15 brain depicting two subcellular segments of layer II/III pyramidal neurons in S1/S2 (modified from Fig. 1c ). (bottom) FACS-sorted GFP-positive cerebrocortical neurons electroporated in utero at E15 and collected at P2 ( Supplementary Fig. S2 ) were immunoblotted for total and acetylated α-tubulin. Depletion of SEPT7 by RNAi caused significant acetylation of α-tubulin. (Triplicated experiments. *** P <0.001 by t -test). Error bars denote s.e.m. ( b , c ) Image-based quantification of acetylated α-tubulin in the somata and dendrites and the axon bundle proximal to the corpus callosum. (top) Representative immunofluorescence images of acetylated α-tubulin in the somata/dendrites ( b ) and in the axon bundle ( c ) of GFP-positive S1/S2 pyramidal neurons with or without SEPT7 depletion via RNAi (#1) or gene disruption. In SEPT7-depleted neurons, microtubules were significantly acetylated in the somata/dendrites and in the axons to a lesser extent. Scale bars, 500 μm ( b ), 200 μm ( c ). Graphs: Acetylated α-tubulin/GFP immunofluorescence ratio in vivo via RNAi (S7KD#1 and #2) or gene disruption (S7KO). All three modes of SEPT7 depletion consistently caused significant acetylation of α-tubulin in the somata/dendrites and in the axons to a lesser extent. (KD; n =12, 6, 6. *** P <0.001 by one-way ANOVA with post hoc Tukey. KO; n =3, *** P <0.001, * P <0.05 by t -test). Error bars denote s.e.m. ( d , e ) Immunoblot estimation of the gross acetylated/total α-tubulin ratio (including GFP-negative untransfected population) in SEPT7-depleted cerebrocortical neurons via RNAi (#1, KD) or gene disruption (KO) at div2. Note that α-tubulin was hyperacetylated in SEPT7-depleted neurons. (Triplicated experiments. * P <0.05, ** P <0.001 by t -test). Error bars denote s.e.m. ( f ) (top) Representative immunofluorescence images of acetylated α-tubulin in pyramidal-like cerebrocortical neurons in culture (div2). The insets show GFP co-expressed with sh Sept7 (#1) or the empty vector. The signals for acetylated α-tubulin were elevated in the soma, dendrites and axons of SEPT7-depleted neurons (SEPT7 KD). Scale bars, 50 μm. (bottom) Quantification of acetylated α-tubulin immunofluorescence measured separately in dendrites and axons, showing that SEPT7 depletion caused hyperacetylation of microtubules in axons and dendrites to a comparable degree. ( n =12, *** P <0.001, ** P <0.01 by t -test). Error bars denote s.e.m. Full size image Consistently, in vitro experiments showed that the amount of acetylated α-tubulin increased after depletion of SEPT7 either via RNAi or gene disruption. In either case, the gross increment of acetylated α-tubulin estimated by immunoblot was 30–40% including the GFP-negative untransfected population ( Fig. 3d,e ; Supplementary Fig. S10 ), whereas the amount of polyglutamylated α-tubulin was changed only by −1% as compared with the control. Immunofluorescence analysis detected hyperacetylated α-tubulin along the dendrites and axons, and in the somata of SEPT7-depleted neurons ( Fig. 3f ). To assess the growth rate of axonal microtubules following SEPT7 depletion, we conducted live imaging of the plus ends of microtubules with GFP-EB1 in div3 (1 day after plating) cerebrocortical neurons from E17 mice. The average anterograde velocity of GFP-EB1 puncta was significantly reduced in the longest neurites (presumed axons) of neurons that co-express sh Sept7 (#1)/mCherry compared with those that express mCherry alone ( Fig. 4a–d ; Supplementary Movies 1 and 2 ). The range of GFP-EB1 velocity in the control group was comparable with the previous results on EB3-GFP in axons [22] , which guarantees the authenticity of our experimental conditions and neuronal viability. These data indicate that the retardation of microtubule growth underlies the stagnant neurite growth after depletion of SEPT7. 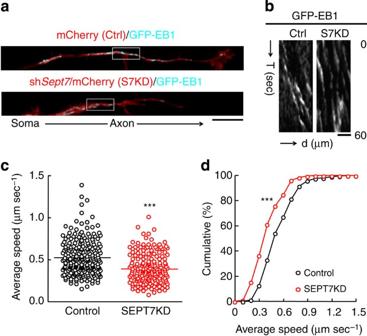Figure 4: Stagnant microtubule growth in SEPT7-depleted cerebrocortical neurons. (a) Representative frames from time-lapse images of GFP-EB1 (cyan), a microtubule plus end tracker, expressed in cerebrocoritical pyramidal-like neurons at div3 (1 day after plating) with or without SEPT7 depletion via RNAi (#1). Each image shows a part of a transfected neuron expressing mCherry whose longest neurite (presumed axon) extends rightward from the soma. Scale bar, 10 μm. (b) Kymographic representation of the anterograde motility of GFP-EB1 puncta. Time-lapse serial images of GFP-EB1 in an axon segment (boxed ina) are stacked. The slope of the trajectory represents the velocity of each GFP-EB1 punctum. Scale bar, 5 μm. (c,d) Anterograde velocity of GFP-EB1 puncta measured in the longest neurites, with or without SEPT7 depletion, and shown as a scattergram (c) and as cumulative curves (d). SEPT7 depletion (S7KD, red) reduced the fast-moving population and shifted the curve to the left. The velocity was measured for 217 (Ctrl) and 188 (S7KD) GFP-EB1 puncta that were tracked for more than 10 s, respectively in 18 and 16 mCherry-expressing neurons that were morphologically comparable. (***P<0.001 byt-test in (c) and by the Kolmogorov–Smirnov test in (d)). Figure 4: Stagnant microtubule growth in SEPT7-depleted cerebrocortical neurons. ( a ) Representative frames from time-lapse images of GFP-EB1 (cyan), a microtubule plus end tracker, expressed in cerebrocoritical pyramidal-like neurons at div3 (1 day after plating) with or without SEPT7 depletion via RNAi (#1). Each image shows a part of a transfected neuron expressing mCherry whose longest neurite (presumed axon) extends rightward from the soma. Scale bar, 10 μm. ( b ) Kymographic representation of the anterograde motility of GFP-EB1 puncta. Time-lapse serial images of GFP-EB1 in an axon segment (boxed in a ) are stacked. The slope of the trajectory represents the velocity of each GFP-EB1 punctum. Scale bar, 5 μm. ( c , d ) Anterograde velocity of GFP-EB1 puncta measured in the longest neurites, with or without SEPT7 depletion, and shown as a scattergram ( c ) and as cumulative curves ( d ). SEPT7 depletion (S7KD, red) reduced the fast-moving population and shifted the curve to the left. The velocity was measured for 217 (Ctrl) and 188 (S7KD) GFP-EB1 puncta that were tracked for more than 10 s, respectively in 18 and 16 mCherry-expressing neurons that were morphologically comparable. (*** P <0.001 by t -test in ( c ) and by the Kolmogorov–Smirnov test in ( d )). Full size image The consistent in vivo and in vitro findings indicate that depletion of SEPT7 from cerebrocortical neurons causes hyperacetylation of microtubules via functional insufficiency of HDAC6. The resulting growth retardation and hyperstabilization ( Supplementary Fig. S6 ) of microtubules [23] are likely to account, at least in part, for the reduced neuritogenesis elicited by the loss of SEPT7. Septins and HDAC6 are associated in vivo and in vitro We reasoned that SEPT7 may promote the deacetylation or suppress the acetylation of α-tubulin via an unknown mechanism. On the basis of previous studies, we tested the possible involvement of the major α-tubulin deacetylase in neurons, HDAC6 (refs 24 , 25 , 26 ). After confirming the expression of HDAC6 in the newborn (P0) cerebral cortices and cerebrocortical neurons at div2–3 ( Fig. 5a,b ; Supplementary Fig. S10 ), we tested whether HDAC6 and septins are associated in extracts of those cells using a co-immunoprecipitation/immunoblot assay. The reciprocal co-immunoprecipitation between subsets of endogenous SEPT7 (in complex with other subunits) and HDAC6 with specific antibodies suggests their physiological association during neuritogenesis ( Fig. 5c and Supplementary Fig. S10 ). To test the association between exogenous SEPT7 and HDAC6, we co-expressed epitope-tagged polypeptides in heterologous cells, and showed that GFP-tagged SEPT7 is captured on anti-Flag antibody-coated beads via Flag-tagged HDAC6 ( Fig. 5d and Supplementary Fig. S10 ). We further tested the direct interaction between the SEPT7-containing septin complex and HDAC6 in vitro . His 6 -tagged SEPT7/6/2 (a canonical septin hetero-oligomer used due to the higher solubility than SEPT7 alone [27] ) that had been expressed in insect cells, then purified and immobilized on beads, captured bacterially expressed recombinant GST-tagged HDAC6 but not GST-tag alone ( Fig. 5e and Supplementary Fig. S10 ). These data collectively support the direct interaction between the SEPT7-containing septin complex and HDAC6. In contrast, the association between SEPT7 and another α-tubulin deacetylase SIRT2 (refs 25 , 26 ), or two major α-tubulin acetyl transferases MEC-17 (ref. 28 ) and ELP3 (ref. 29 ), was not detectable in cerebrocortical neurons ( Supplementary Fig. S7 ). 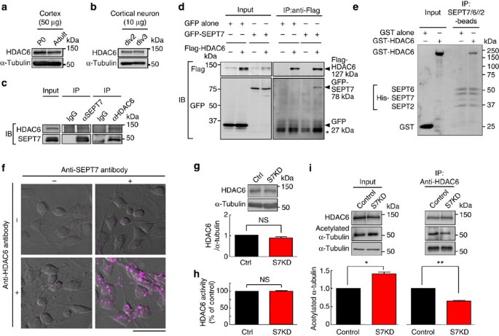Figure 5: Physiological and direct interaction between septins and the major tubulin deacetylase HDAC6. (a,b) Immunoblot for endogenous HDAC6 (a) in newborn (P0) and adult cerebral cortex and (b) in primary cerebrocortical neurons at div2 and 3. Each lane respectively contained 50/10 μg total protein. (c) Mutual co-immunoprecipitation of endogenous SEPT7 and HDAC6. Lysates from div2 cerebrocortical neurons were incubated with protein A beads coated with nonimmune IgG, anti-SEPT7 antibody or anti-HDAC6 antibody, and these proteins were detected by immunoblot in a reciprocal manner. (d) Co-expression and mutual co-immunoprecipitation of GFP-SEPT7 and Flag-HDAC6 in heterologous cells. (Left) Anti-Flag antibody detected Flag-HDAC6 (and gave nonspecific faint bands in the 1st and 3rd lanes) and anti-GFP antibody detected GFP and GFP-SEPT7. (Right) When Flag- HDAC6 was captured on anti-Flag beads, GFP-SEPT7 was co-immunoprecipitated, but GFP was not (compare the 2nd and 4th lanes. *, IgG light chain). (e) Direct binding between the purified, recombinant septin complex and HDAC6in vitro. Immobilized His-tagged SEPT7/6/2 captured GST-HDAC6 but not GST alone. (Coomassie blue staining). (f) Representative results ofin situproximity ligation assay for endogenous SEPT7 and HDAC6 in div2 cerebrocortical neurons. Fluorescent puncta were generated in the somata and neurites only when anti-SEPT7 antibodies and anti-HDAC6 antibodies were present in close proximity. Scale bars, 25 μm. (g) Immunoblot showing that SEPT7 depletion did not affect the amount of HDAC6 in div2 cerebrocortical neurons. (Triplicated experiment. NS,P>0.05 byt-test). Error bars denote s.e.m. (h) SEPT7 depletion via RNAi (#1, S7KD) did not alter the deacetylating activity of HDAC6. Cell lysates as in (b) were subjected to anin vitroassay with a fluorogenic substrate. (Triplicated experiment. NS,P>0.05 byt-test). Error bars denote s.e.m. (i) SEPT7 depletion via RNAi (#1, S7KD) caused dissociation of HDAC6 and acetylated α-tubulin. (Left) Cell lysates as in (b,h) were immunoblotted for endogenous HDAC6, acetylated α-tubulin and total α-tubulin. Hyperacetylation of α-tubulin in SEPT7-depleted neurons was recapitulated (cf.Fig. 3d). Each lane contained 50 μg total protein. (Right) Although SEPT7 depletion increased acetylated α-tubulin, its association with HDAC6 was paradoxically reduced. (Triplicated experiments. *P<0.05, **P<0.01 byt-test). Error bars denote s.e.m. Figure 5: Physiological and direct interaction between septins and the major tubulin deacetylase HDAC6. ( a , b ) Immunoblot for endogenous HDAC6 ( a ) in newborn (P0) and adult cerebral cortex and ( b ) in primary cerebrocortical neurons at div2 and 3. Each lane respectively contained 50/10 μg total protein. ( c ) Mutual co-immunoprecipitation of endogenous SEPT7 and HDAC6. Lysates from div2 cerebrocortical neurons were incubated with protein A beads coated with nonimmune IgG, anti-SEPT7 antibody or anti-HDAC6 antibody, and these proteins were detected by immunoblot in a reciprocal manner. ( d ) Co-expression and mutual co-immunoprecipitation of GFP-SEPT7 and Flag-HDAC6 in heterologous cells. (Left) Anti-Flag antibody detected Flag-HDAC6 (and gave nonspecific faint bands in the 1st and 3rd lanes) and anti-GFP antibody detected GFP and GFP-SEPT7. (Right) When Flag- HDAC6 was captured on anti-Flag beads, GFP-SEPT7 was co-immunoprecipitated, but GFP was not (compare the 2nd and 4th lanes. *, IgG light chain). ( e ) Direct binding between the purified, recombinant septin complex and HDAC6 in vitro . Immobilized His-tagged SEPT7/6/2 captured GST-HDAC6 but not GST alone. (Coomassie blue staining). ( f ) Representative results of in situ proximity ligation assay for endogenous SEPT7 and HDAC6 in div2 cerebrocortical neurons. Fluorescent puncta were generated in the somata and neurites only when anti-SEPT7 antibodies and anti-HDAC6 antibodies were present in close proximity. Scale bars, 25 μm. ( g ) Immunoblot showing that SEPT7 depletion did not affect the amount of HDAC6 in div2 cerebrocortical neurons. (Triplicated experiment. NS, P >0.05 by t -test). Error bars denote s.e.m. ( h ) SEPT7 depletion via RNAi (#1, S7KD) did not alter the deacetylating activity of HDAC6. Cell lysates as in ( b ) were subjected to an in vitro assay with a fluorogenic substrate. (Triplicated experiment. NS, P >0.05 by t -test). Error bars denote s.e.m. ( i ) SEPT7 depletion via RNAi (#1, S7KD) caused dissociation of HDAC6 and acetylated α-tubulin. (Left) Cell lysates as in ( b , h ) were immunoblotted for endogenous HDAC6, acetylated α-tubulin and total α-tubulin. Hyperacetylation of α-tubulin in SEPT7-depleted neurons was recapitulated ( cf. Fig. 3d ). Each lane contained 50 μg total protein. (Right) Although SEPT7 depletion increased acetylated α-tubulin, its association with HDAC6 was paradoxically reduced. (Triplicated experiments. * P <0.05, ** P <0.01 by t -test). Error bars denote s.e.m. Full size image To visualize the subcellular location where SEPT7 and HDAC6 associate, we used the in situ proximity ligation assay (PLA) [30] for sprouting cerebrocortical neurons in culture. In theory, a pair of antibodies that recognize endogenous SEPT7 and HDAC6 in close proximity (<40 nm) mediates a local enzymatic reaction that generates a submicron fluorescent deposit. The fluorescent puncta, which represent antibody-crosslinked SEPT7 and HDAC6, were distributed both in the soma and neurite ( Fig. 5f ). Taken together, the physical interaction between the SEPT7–containing septin complex and HDAC6 was consistently detected in biochemical assays and was corroborated by their proximity in situ . SEPT7 facilitates HDAC6/acetylated α-tubulin interaction Given the direct molecular interaction between septins and HDAC6, and between HDAC6 and acetylated α-tubulin as a substrate, a simple mechanism connecting the depletion of SEPT7 to microtubule hyperacetylation could involve the collateral depletion and/or inhibition of HDAC6. However, this scheme seems unlikely, as depletion of SEPT7 did not significantly alter the amount of HDAC6 or its enzymatic activity on a fluorogenic substrate ( Fig. 5g,h ; Supplementary Figs S8 and S10 ). Intriguingly, despite the accumulation of acetylated α-tubulin in SEPT7-depleted cells ( Fig. 3d,e ), the HDAC6-bound fraction of acetylated α-tubulin was paradoxically reduced ( Fig. 5i and Supplementary Fig. S10 ). This discordance indicates a reduced accessibility of HDAC6 to acetylated α-tubulin in the absence of SEPT7, and favours another scheme: Interaction with the septin complex may enhance the accessibility of HDAC6 to acetylated α-tubulin, possibly by hindering the access of competitive binding partners that include substrates of HDAC6. Inhibition of HDAC6 gives a phenocopy of SEPT7 depletion To probe the functional interaction between SEPT7 and HDAC6, we tested whether inhibiting microtubule deacetylation by HDAC6 could mimic and/or synergize the effect of SEPT7 depletion on neuritogenesis of cerebrocortical neurons in vitro . The deacetylation activity of HDAC6 was directly inhibited by a selective, cell-permeable HDAC6 inhibitor, tubacin ( tub ulin ac etylation in ducer) [31] . Treatment of cerebrocortical neurons with 10 μM tubacin (from 6 h after plasmid transfection through to div2) significantly increased the level of acetylated α-tubulin without altering the level of total α-tubulin, raising the acetylated/total α-tubulin ratio by 34%. Morphometry, scattergram and statistical analyses revealed that tubacin suppressed the growth of both dendrites and axons more potently than did the depletion of SEPT7 via RNAi (#1), and the combination of those two genetic/chemical techniques did not give additive effects ( Fig. 6a–e ). The potent inhibition of neuritogenesis by tubacin corroborates that HDAC6 is the critical α-tubulin-deacetylating enzyme in sprouting cerebrocortical neurons. 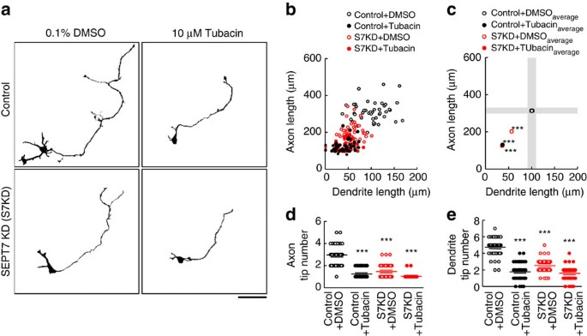Figure 6: Direct inhibition of HDAC6 by tubacin gives a phenocopy of SEPT7 depletion. (a) (Top panels) Representative images of GFP-expressing cerebrocortical neurons at div2 treated with vehicle alone (0.1% DMSO) or with 10 μM tubacin in vehicle. HDAC6 inhibition by tubacin inhibited the growth of both dendrites and axons. (Bottom panels) SEPT7 depletion via RNAi (#1) combined with tubacin treatment did not exhibit an obvious additive effect on neurite morphology. Scale bar, 50 μm. (b) Scattergram of total dendrite length and total axon length of pyramidal-like cerebrocortical neurons treated with tubacin and SEPT7-depletion in the four combinations shown in (a). The growth of both dendrites and axons was markedly inhibited by tubacin treatment (black closed circles) in comparison with the control (black open circles), which was not enhanced by additional depletion of SEPT7 (red closed circles). (c) Statistical analysis of the results shown in (b) with plots of the mean values, showing that tubacin treatment significantly and proportionally shortened dendrites and axons. The neurite-shortening effect of tubacin was more potent than, and not enhanced by, SEPT7 depletion. The grey bars represent average±2 s.e.m. of the control samples. (n=45 × 4. ***P<0.001 by one-way ANOVA withpost hocTukey). Error bars denote s.e.m. (dande) Tip numbers of axons and dendrites in the above samples were significantly reduced by tubacin alone, by SEPT7 depletion alone, or by the combination of the two. (n=45 × 4. ***P<0.001 by one-way ANOVA withpost hocTukey). Error bars denote s.e.m. Figure 6: Direct inhibition of HDAC6 by tubacin gives a phenocopy of SEPT7 depletion. ( a ) (Top panels) Representative images of GFP-expressing cerebrocortical neurons at div2 treated with vehicle alone (0.1% DMSO) or with 10 μM tubacin in vehicle. HDAC6 inhibition by tubacin inhibited the growth of both dendrites and axons. (Bottom panels) SEPT7 depletion via RNAi (#1) combined with tubacin treatment did not exhibit an obvious additive effect on neurite morphology. Scale bar, 50 μm. ( b ) Scattergram of total dendrite length and total axon length of pyramidal-like cerebrocortical neurons treated with tubacin and SEPT7-depletion in the four combinations shown in ( a ). The growth of both dendrites and axons was markedly inhibited by tubacin treatment (black closed circles) in comparison with the control (black open circles), which was not enhanced by additional depletion of SEPT7 (red closed circles). ( c ) Statistical analysis of the results shown in ( b ) with plots of the mean values, showing that tubacin treatment significantly and proportionally shortened dendrites and axons. The neurite-shortening effect of tubacin was more potent than, and not enhanced by, SEPT7 depletion. The grey bars represent average±2 s.e.m. of the control samples. ( n =45 × 4. *** P <0.001 by one-way ANOVA with post hoc Tukey). Error bars denote s.e.m. ( d and e ) Tip numbers of axons and dendrites in the above samples were significantly reduced by tubacin alone, by SEPT7 depletion alone, or by the combination of the two. ( n =45 × 4. *** P <0.001 by one-way ANOVA with post hoc Tukey). Error bars denote s.e.m. Full size image Taken together, we conclude that the functional insufficiency, without inhibiting the enzymatic activity, of HDAC6 underlies the short neurite phenotype found in SEPT7-depleted neurons, and that HDAC6-mediated modification of microtubules is a major biochemical process that connects the gap between the loss of SEPT7 and neuritogenesis defects in vivo and in vitro . In this study, we provide the most compelling evidence to date demonstrating the cell autonomous requirement of the septin subunit SEPT7 for dendrite growth and terminal extension/branching of axons of cerebrocortical neurons in pre- and postnatal mouse brain development. The results were consistent regardless of the means used to deplete SEPT7 (RNAi and conditional Sept7 gene disruption) and of the system ( in vivo and in vitro ). Biochemical, pharmacological and imaging analyses uncovered that septins/HDAC6-mediated deacetylation of microtubules is the common mechanism that couples septins and the dynamic growth of microtubules, shared by the dendrites and axons of sprouting neurons ( Fig. 7 ). 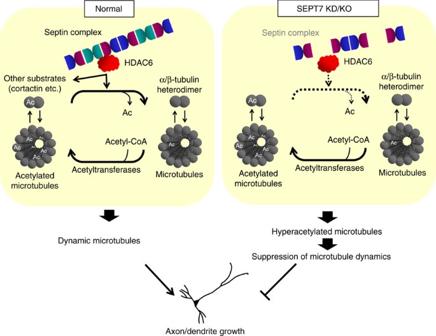Figure 7: Schematic diagram illustrating the involvement of the HDAC6-septin association in microtubule deacetylation and axon/dendrite growth. HDAC6 is the major microtubule deacetylase, which promotes microtubule remodelling by counteracting acetyl transferases that stabilize microtubules55. This study demonstrated that the direct interaction with the septin complex facilitates the access of HDAC6 to acetylated α-tubulin and/or stabilizes the enzyme-substrate interaction without altering the deacetylation activity of HDAC6. An open question is whether the putative tripartite interaction of the septin complex/HDAC6/acetylated α-tubulin (a subset of the signals in the PLA assay shown inFig. 5fshould represent this) occurs on α/β-tubulin heterodimers, protofilaments and/or microtubules. It is also worth testing whether an actomyosin-dependent mechanism, including another HDAC6 substrate cortactin16, could contribute to the stagnant neurite growth after septin depletion. Independent of the specific underlying mechanism, the novel molecular network identified in this study has shed new light on the common machinery for the growth of axons and dendritesin vivoandin vitro. Figure 7: Schematic diagram illustrating the involvement of the HDAC6-septin association in microtubule deacetylation and axon/dendrite growth. HDAC6 is the major microtubule deacetylase, which promotes microtubule remodelling by counteracting acetyl transferases that stabilize microtubules [55] . This study demonstrated that the direct interaction with the septin complex facilitates the access of HDAC6 to acetylated α-tubulin and/or stabilizes the enzyme-substrate interaction without altering the deacetylation activity of HDAC6. An open question is whether the putative tripartite interaction of the septin complex/HDAC6/acetylated α-tubulin (a subset of the signals in the PLA assay shown in Fig. 5f should represent this) occurs on α/β-tubulin heterodimers, protofilaments and/or microtubules. It is also worth testing whether an actomyosin-dependent mechanism, including another HDAC6 substrate cortactin [16] , could contribute to the stagnant neurite growth after septin depletion. Independent of the specific underlying mechanism, the novel molecular network identified in this study has shed new light on the common machinery for the growth of axons and dendrites in vivo and in vitro . Full size image Previously, the functional role(s) of septins in neurons had remained controversial: RNAi in cultured neurons gave morphological phenotypes such as dendrite malformation of rat hippocampal neurons [14] , [15] or aberrant axon branching of chick dorsal root ganglia neurons [16] . In contrast, no gross neuroanatomical deficit was reported in conventional knockout mice that lack SEPT3, 4, 5, 6, 3+5 or 4+6 (refs 7 , 8 , 9 , 10 , 11 ). This led to the notion that perhaps septins might be dispensable as cytoskeletal or structural components in neurons, but that septins might rather compartmentalize and/or coordinate proper targeting/complexing of signalling molecules and transporters [10] , [32] , [33] , [34] . Our observations indicating that SEPT7 facilitates the access of HDAC6 to acetylated α-tubulin reconcile the seemingly contradictory observations and underscore the critical role of septins as a scaffold for microtubule regulation. A previous study with the dog kidney-derived MDCK cell line showed that the non-neuronal septin subunit SEPT2 is associated with polyglutamylated microtubules [35] , a subset of which is required to guide microtubule growth [36] . However, in cerebrocortical neurons, the amount of polyglutamylated α-tubulin changed only by −1% after the depletion of SEPT7. In HeLa cells, depletion of SEPT7 or SEPT2 releases a septin binding partner, MAP4, and the resulting relocation of MAP4 causes hyperstabilization of microtubules [37] . In neurons, however, MAP4 is much lower in abundance than the major microtubule-associated proteins, MAP2 and tau. Thus, the previously reported molecular mechanisms that mediate septins and microtubules in heterologous cells are unlikely to have major roles in neuritogenesis. The physical interaction between septins and HDAC6 is consistent in three distinct biochemical assays; first, co-immunoprecipitation of native SEPT7 and HDAC6 from extracts of cerebrocortical neurons; second, co-immunoprecipitation of SEPT7 and HDAC6 co-expressed in nonneural cells; and finally, beads-capture assay with a pure recombinant SEPT7/6/2 complex and HDAC6. SEPT7–HDAC6 interaction was less obvious in the first than in second or third assay, implying that the interaction is subject to their biochemical states (for example, post-translational modifications of HDAC6 and the composition of septin hetero-oligomers) and/or the environment (for example, competition with other interaction partners expressed in neurons). HDAC6, which belongs to a class II histone deacetylase family, is a multidomain deacetylase/adaptor protein with tandem catalytic domains and a ubiquitin-binding zinc finger. HDAC6 interacts with and exerts pleiotropic effects on or with diverse proteins, which are categorized into at least two classes; (1) deacetylation substrates (for example, α-tubulin, HSP90, cortactin), and (2) adapters (for example, β-tubulin, p150 glued /dynactin, Cdc20, polyubiquitin) [38] . Given the multiple binding partners of HDAC6 and the fact that depletion of SEPT7 reduces HDAC6-bound acetylated α-tubulin without affecting HDAC6 activity in neurons, a simple hypothesis would be that septins facilitate the interaction between acetylated α-tubulin and HDAC6 by hindering the access of competing binding partners or substrates to HDAC6. This model may account for the requirement of septins to maintain microtubule dynamics for neurite growth through HDAC6-mediated deacetylation. That model is supported by the facts that another α-tubulin deacetylase SIRT2 (refs 25 , 26 ), acetyltransferase elongator complex components MEC-17 (ref. 28 ) and ELP-3 (ref. 29 ) do not interact with SEPT7, and that their amounts do not change by depletion of SEPT7 ( Supplementary Fig. S7 ), although other possibilities are not excluded. This study has disclosed a novel molecular link integrating septins, microtubules and HDAC6, a critical protein-modifying enzyme that couples the two cytoskeletal systems for the coordination of neurite growth during brain development. As several septin subunits are significantly accumulated in postmortem human brains with psychiatric disorders [39] and Hdac6 -null mice exhibit hyperactivity and resistance against anxiety/depression [40] , [41] , [42] , post-developmental function and neuropathological involvement of the septin-HDAC6-microtubule axis await further examination. Previous studies have demonstrated that Hdac6 -null mice do not develop an obvious brain anomaly [40] , and that genetic or chemical inhibition of HDAC6 delays the progression of mouse models of adult-onset neurodegeneration, for example, Charcot-Marie-Tooth disease ( HSPB1 −/− ) [43] and amyotrophic lateral sclerosis ( SOD1 G93A ) [44] . However, it remains unclear whether an HDAC6-targeting therapeutic regimen would be beneficial in the context of the developing brain and in adult neurogenesis, because acute depletion of HDAC6 via RNAi causes severe defects in dendritogenesis and axonogenesis in vitro and in vivo [45] , [46] . Our present study, which aimed at understanding the role of SEPT7, has provided further evidence for the developmental stage-specific requirement of HDAC6 in early neuritogenesis, and uncovered the SEPT7-HDAC6-microtubule axis as a novel molecular mechanism underlying neurite development. As the neuritogenesis phenotype was more pronounced through acute HDAC6 inhibition than through acute SEPT7 depletion ( Fig. 6 ), future studies must address whether some forms of initial neuritogenesis defects may have been obscured by compensation in the Hdac6 -null mice. Considering the physical and functional interaction between septins and HDAC6 in mammalian neurons, pleiotropic phenotypes caused by the loss or excess of septins could be attributed partly to HDAC6 insufficiency or dysregulation, and vice versa. For instance, the loss of SEPT4 in mice diminishes resistance against α-synuclein toxicity and dopaminergic function [10] , whereas HDAC6 protects Drosophila dopamine neurons from α-synuclein toxicity [47] . Future studies along these lines should help elucidate the composite dysregulation of septins, HDAC6 and microtubules that may underlie the pathophysiology of developmental, psychiatric and neurodegenerative disorders in humans. Plasmid constructions One of the RNAi vectors used, pmU6pro-SEPT7, had been designed for the targeting of nucleotides 1005–1024 (#2) of mouse Sept7 (ref. 27 ). The other RNAi vectors targeting nucleotides 1175–1196 (#1) were constructed in UI4_GFP_SIBR or UI4_mCherry_SIBR [20] , each of which co-expresses shRNA and GFP or mCherry. The RNAi-resistant SEPT7 mutant (SEPT7res) was generated by introducing silent mutations into the sequence #1 in pEGFP-SEPT7 (ref. 15 ), which was transferred into the pmCherry vector (a gift from Dr R.Y. Tsien at UCSD/HHMI [48] ) to generate pmCherry-SEPT7res. Plasmids for a Flag-tagged HDAC6 (#13823) and a Myc-tagged Cre (#13775) were obtained from Addgene. Animal experiments and establishment of Sept7 fl/fl mice Animal experiments were approved by the Institutional Review Committee and conducted in accordance with the regulations for the care and use of experimental animals at Nagoya University. Conditional targeting of Sept7 (exon 3) was conducted by homologous recombination with C57BL/6-derived Bruce 4 embryonic stem cells, verified by Southern blot and PCR of genomic DNA. Myc-tagged Cre was introduced into Sept7 fl/fl neurons via electroporation. The recombination and SEPT7 protein decay were verified by PCR and immunoblot assays, respectively. This mouse line has been deposited to RIKEN Bioresource Center (RBRC05390). In vivo assays In utero electroporation was conducted by injecting a mixture of UI4_GFP_SIBR- or pmU6pro-derived constructs (for Sept7 +/+ embryos) or Myc-Cre (for Sept7 fl/fl embryos), plus pCAG-EGFP and 0.05% Fast Green (tracer) into the lateral ventricles of embryos at E12/15. Pregnant mice were anaesthetized with intraperitoneal injection of sodium pentobarbital (50 μg g −1 , Nembutal, Abbott Laboratories) in saline. Embryos were approached through the uterus pulled out from midline laparotomy. Glass capillary tubes (GC150TF-10; Harvard Apparatus) were tapered using a micropipette puller (Narishige). One microliter of plasmid solution (0.5–1.0 g l −1 ) was injected into the right lateral ventricle of each embryo, and 5 square electric pulses (50 mV, 50 msec) were given in 5 sec with an electroporator (CUY21EDIT; NepaGene) [19] . Serial sagittal sections of the upper spinal cord (30 μm-thick) and/or serial coronal brain sections (50 μm-thick) were prepared at P1/14/15/30. Quantitative image analyses, including the morphology-based identification of axons/dendrites ( Supplementary Fig. S9 ), were conducted by using software MetaMorph (6.3r7, Molecular Devices). For the measurement of dendrites in the brain, GFP-positive dendrites from pyramidal neurons in the layer II/III of S1/S2 were traced in 1 μm-thick serial confocal sections. After assigning all dendrites to each soma, their total lengths projected onto a two-dimensional plane were measured. FACS analysis Six days after in utero electroporation of plasmids for RNAi, cerebral cortical tissues of P2 pups (mixed sex) were dissected and dispersed with an enzyme-free cell dissociation buffer (GIBCO). A flow cytometer (FACS Aria2, BD) was used to collect well-separated, propidium iodide-negative (viable), and GFP-positive cells. Cell culture Cerebrocortical neurons from embryos were prepared and cultured using an established protocol [19] , [49] . Briefly, dissected cerebral cortices were incubated for 10 min with 10 g l −1 trypsin type XI (Sigma) plus 0.5 g l −1 DNase I type IV (Sigma) at room temperature and mechanically dissociated in Hanks solution (pH 7.4) (Sigma) with 0.5 g l −1 DNase I type IV and 12 mM MgSO 4 . Dissociated cells were transfected immediately by electroporation using Nucleofector (Amaxa Biosystems) and plated onto 12 mm poly- L -lysine-coated coverslips at the density of 7.5 × 10 5 cells per coverslip in 24-well plates (Greiner) containing minimum essential medium (Invitrogen) with 5 g l −1 glucose, 0.2 g l −1 NaHCO 3 , 0.1 g l −1 transferrin (Calbiochem), 2 mM GlutaMAX-I (Invitrogen), 25 mg l −1 insulin (Sigma), 1 × B-27 supplement (Invitrogen), and 10% fetal bovine serum. Tubacin [31] or nocodazole (Sigma), 10 μM each, was added to the medium 6 h after plating. HEK293T and N-18 cells [50] were grown in Dulbecco's modified Eagle's medium supplemented with 10% fetal bovine serum. Cultures were maintained in 5% CO 2 at 37 °C. Immunocytochemisty and immunohistochemistry Cultured neurons and brain tissues were immunostained after with 4% paraformaldehyde/PBS, permeabilization with 0.1% Triton X-100/PBS, and blocking with 2% BSA/PBS [19] , [49] . We used commercial antibodies as follows: rat or rabbit anti-GFP (1:1,000, Nacalai or Molecular Probes), rabbit anti-DsRed (1:1,000, Clontech); mouse anti-tau-1 (1:1,000, Millipore), anti-neurofilament smi312 (1:2,000, Covance), anti-MAP2 (1:1,000, Chemicon), anti-Myc (1:1,000), anti-acetylated α-tubulin (1:1,000), and anti-α-tubulin (1:4000) (Sigma). We used the original affinity-purified rabbit polyclonal antibodies, anti-SEPT7 (1:4,000) [10] and anti-HDAC6 (epitope: mouse HDAC6 1137–1149 ) (1 mg l −1 ). For secondary antibodies, we used Alexa 405-, 488-, 555-, 568-, 594- or 633-conjugated antibodies against rabbit, and mouse or rat immunoglobulin (Ig) Gs (1:250–1,000, Molecular Probes). Fluorescence imaging was conducted using scanning laser confocal microscopes IX81/FV1000 (Olympus) with a × 40 objective lens (NA 1.0) and LSM-780 (Zeiss) with × 40 (NA 1.1) and × 63 (NA 1.4) objective lenses, and wide-field microscopes (BZ-9000, Keyence or BX-60, Olympus) with × 40 and × 20 objective lenses (NA 1.3, Nikon or NA 0.7, Olympus). Image acquisition and morphometric analyses in vitro For the accurate tracing of neurites, transfected and untransfected cells were mixed at a ratio of 1:10, grown in vitro for two days, fixed and immunostained for morphometry as follows. Pyramidal-like neurons that bore one unambiguously recognizable axon and one or more dendrites were analysed. For each neuron, the axon was discriminated from dendrites by tau-1 staining and/or an established morphological criteria (that is, relative length, diameter and position) [19] , [49] . Axon and dendrite lengths, and branch tip numbers were measured manually using an ImageJ plugin, NeuronJ 1.1.0 (ref. 51 ) by an observer blinded to the identity of the samples. Live imaging Cerebrocortical neurons co-transfected with GFP-EB1 (ref. 52 ) and sh Sept7 /mCherry or mCherry by electroporation were incubated in suspension for 2 days, then plated at a density of 10 6 in glass-bottom culture dishes (MatTek). At div3 (1 day after plating), the culture medium was replaced with Tyrode solution (129 mM NaCl, 5 mM KCl, 2 mM CaCl 2 , 2 mM MgCl 2 , 30 mM D -glucose, 25 mM Hepes, pH 7.4). The cells on a stage incubator at 37 °C were imaged using an LSM-780 microscope with a × 63 objective lens at a rate of 1 s per frame for 400 s. We randomly selected seven neurons from those that met morphological criteria, and measured the velocity of all GFP-EB1 puncta that were unambiguously tracked for >10 s. The movie files were reconstructed with ImageJ and the kymograph plugin was additionally used. In situ PLA The proximity between HDAC6 and SEPT7 in cultured neurons was assessed by in situ PLA [30] using the Duolink In Situ Red kit (Olink Bioscience). The anti-SEPT7 and anti-HDAC6 antibodies were linked, respectively, to the plus and minus PLA probes, and were incubated with fixed neurons for 16 h at 4 °C. After washing, the samples were further processed to assess whether the two antigens were close enough (<40 nm) to generate fluorescent signals. Microtubule stability assay A standard nocodazole-based microtubule stability assay [53] was used with cultured mouse N-18 neural cells. Briefly, 2 days after transfection of either UI4_GFP_SIBR-SEPT7 or the cognate empty vector, cells were treated with nocodazole (10 μM) for 1 h, fixed with cold methanol and immunostained for α-tubulin. Randomly sampled cells were line-scanned across the long axis for α-tubulin immunofluorescence. Immunoblotting Samples were lysed with brief sonication in Laemmli’s buffer. Polypeptides were resolved by 8 or 10% SDS-PAGE and were transferred onto reinforced nitrocellulose or polyvinylidene difluoride membranes, which were blocked with 5% skim milk in TBST (100 mM Tris-HCl, pH 7.4, 150 mM NaCl, 0.05% Tween-20) and blotted with primary antibodies. Densitometric detection of chemiluminescence was conducted with anti-rabbit or -mouse IgG (Jackson) ECL-Plus reagent (Perkin Elmer), TrueBlot anti-mouse or rabbit Ig (Rockland Immunochemicals), and an image analyser LAS-3000mini (Fuji). Immunoprecipitation Dispersed neurons electroporated with UI4_GFP_SIBR-SEPT7 or the control plasmid were assayed at div3. HEK293T cells (10 6 ) were transfected with FuGENE6 (Roche Diagnostics) to introduce the following plasmids (0.5 μg each), pEGFP, pEGFP-SEPT7 (ref. 50 ), Flag (Sigma) or Flag-HDAC6. Two days later, the cells were lysed in a buffer (10 mM Tris-HCl at pH 7.4, 150 mM NaCl, 1% Triton X-100), centrifuged and the supernatant was mixed with protein G or A-magnetic beads (New England Biolabs) preincubated with mouse anti-FLAG M2 (Sigma), rabbit anti-HDAC6 (ref. 54 ), mouse anti-SIRT2 (Santa Cruz), rabbit anti-MEC-17 (LSBio), rabbit anti-ELP3 (Cell Signaling) or rabbit anti-SEPT7 (ref. 10 ). Immune complexes on the beads were analysed by immunoblot. In vitro binding assay Sf9-expressed His 6 -tagged SEPT7/6/2 (ref. 27 ) was immobilized on Ni-NTA beads (Qiagen) and incubated with Sf9-expressed GST-tagged human HDAC6 (SignalChem) or GST alone in PBS for 6 h at 4 °C. The beads were extensively washed with PBS, and subjected to SDS-PAGE and Coomassie blue staining. Enzymatic activity measurement for HDAC6 A fluorogenic HDAC6 assay kit (BPS Bioscience) and a fluorescence microplate reader (EnSpire, Perkin Elmer) were used to measure the fluorescence intensity of a deacetylated small molecule substrate, which was incubated with each sample in 50 μl at 37 °C for 0.5 h. Statistical analyses Quantitative data are shown as means±s.e.m. Prism 4.0 (GraphPad Software) was used for statistical analyses. T -test and one-way ANOVA with post hoc Tukey test were respectively applied for comparisons between two groups and three groups or more. How to cite this article: Ageta-Ishihara, N. et al. Septins promote dendrite and axon development by negatively regulating microtubule stability via HDAC6-mediated deacetylation. Nat. Commun. 4:2532 doi: 10.1038/ncomms3532 (2013).